Inducing a direct-to-pseudodirect bandgap transition in wurtzite GaAs nanowires with uniaxial stress Many efficient light-emitting devices and photodetectors are based on semiconductors with, respectively, a direct or indirect bandgap configuration. The less known pseudodirect bandgap configuration can be found in wurtzite (WZ) semiconductors: here electron and hole wave-functions overlap strongly but optical transitions between these states are impaired by symmetry. Switching between bandgap configurations would enable novel photonic applications but large anisotropic strain is normally needed to induce such band structure transitions. Here we show that the luminescence of WZ GaAs nanowires can be switched on and off, by inducing a reversible direct-to-pseudodirect band structure transition, under the influence of a small uniaxial stress. For the first time, we clarify the band structure of WZ GaAs, providing a conclusive picture of the energy and symmetry of the electronic states. We envisage a new generation of devices that can simultaneously serve as efficient light emitters and photodetectors by leveraging the strain degree of freedom. In semiconductors, efficient light emission occurs when two conditions are met: the electron and the hole wavefunctions must overlap strongly in the wave-vector space, and the symmetry of the states involved in the radiative process must be compatible with the dipole transitions [1] . Semiconductors with a direct bandgap configuration, such as zincblende (ZB) GaAs, fulfill both conditions and have empowered the photonic and optoelectronic industries [2] . Indirect bandgap semiconductors, such as silicon or germanium, also have electron and hole states at the centre of the Brillouin zone, whose symmetry is compatible with light emission. However, electrons occupy lower-energy states at the edge of the Brillouin zone, causing a reduction of the overlap with the hole wavefunction, which suppresses the light emission. To realize nano-photonic devices directly integrated on silicon, considerable efforts have been made to induce a direct bandgap configuration in indirect bandgap semiconductors like germanium. However, the fact that an anisotropic strain of more than 4% is needed to induce such a transition hampers the development of such photonic applications [3] , [4] , [5] , [6] , [7] . By reducing the semiconductor dimensions down to the nanowire geometry, high levels of strain can be accommodated and enable novel degrees of freedom for the control of the band structure [8] , [9] , [10] , [11] . Precise control of the morphology [12] and crystal structure [13] have made it possible to grow pure single-crystal wurtzite (WZ) nanowires, not available in bulk or thin-film form [14] , [15] . WZ crystals are characterized by a peculiar band structure, shown in Fig. 1 : the heavy, light and split-off holes are non-degenerate at the Γ-point and the conduction band consists of two states. One corresponds to the conduction band of ZB crystals and is indicated as the ‘bright’ conduction band (symmetry Γ 7 c in double group notation, shown in green), whereas the other is related to the states found at the L-point in ZB and is indicated as the ‘dark’ conduction band (symmetry Γ 8 c in double group notation, shown in orange) [16] , [17] . 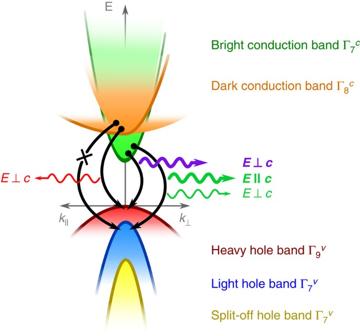Figure 1: Band structure and symmetry of the states for wurtzite GaAs. The conduction band consists of the bright conduction band (Γ7csymmetry, indicated in green) and the dark conduction band (Γ8csymmetry, indicated in orange). The effective mass of the dark conduction band is expected to be highly anisotropic and higher in thec-axis direction (left side of the momentum axis, indicated byk||). The valence band is constituted by the heavy-hole band (symmetry Γ9v, shown in red), the light-hole band and the crystal-field split-off hole band (both with symmetry Γ7v, indicated in blue and yellow, respectively). The symmetries at the Γ-point are given in WZ double-group notation28, that is, including the spin–orbit interaction. Optical transitions between conduction and valence bands are indicated by black arrows connecting the bands involved, and by coloured arrows indicating the photon emitted and its polarization. Bold polarization labels and thick arrows indicate that the transition is allowed even if the spin–orbit interaction is disregarded (in the WZ point group notation), whereas thin polarization labels and arrows indicate that the corresponding transition is allowed only if the spin–orbit interaction is taken into consideration (in the WZ double group notation) and the corresponding oscillator strength is expected to be small35. Radiative processes between the bright Γ7cconduction band and all valence band states are possible: transitions into the heavy-hole states (represented in purple) are expected to have polarization orthogonal to the nanowire’sc-axis; transitions into the light-hole states (represented in green) are expected to be strongly polarized along the nanowire’sc-axis, but also have a small perpendicular component. The optical transitions from the dark Γ8cconduction band are possible only if spin–orbit effects are taken into account. In particular, the transition (represented in red) between the dark conduction band and the heavy-hole state is expected to have a polarization perpendicular to the nanowire’sc-axis. Transitions with the light-hole state are always forbidden (indicated by a cross). Figure 1: Band structure and symmetry of the states for wurtzite GaAs. The conduction band consists of the bright conduction band (Γ 7 c symmetry, indicated in green) and the dark conduction band (Γ 8 c symmetry, indicated in orange). The effective mass of the dark conduction band is expected to be highly anisotropic and higher in the c -axis direction (left side of the momentum axis, indicated by k || ). The valence band is constituted by the heavy-hole band (symmetry Γ 9 v , shown in red), the light-hole band and the crystal-field split-off hole band (both with symmetry Γ 7 v , indicated in blue and yellow, respectively). The symmetries at the Γ-point are given in WZ double-group notation [28] , that is, including the spin–orbit interaction. Optical transitions between conduction and valence bands are indicated by black arrows connecting the bands involved, and by coloured arrows indicating the photon emitted and its polarization. Bold polarization labels and thick arrows indicate that the transition is allowed even if the spin–orbit interaction is disregarded (in the WZ point group notation), whereas thin polarization labels and arrows indicate that the corresponding transition is allowed only if the spin–orbit interaction is taken into consideration (in the WZ double group notation) and the corresponding oscillator strength is expected to be small [35] . Radiative processes between the bright Γ 7 c conduction band and all valence band states are possible: transitions into the heavy-hole states (represented in purple) are expected to have polarization orthogonal to the nanowire’s c -axis; transitions into the light-hole states (represented in green) are expected to be strongly polarized along the nanowire’s c -axis, but also have a small perpendicular component. The optical transitions from the dark Γ 8 c conduction band are possible only if spin–orbit effects are taken into account. In particular, the transition (represented in red) between the dark conduction band and the heavy-hole state is expected to have a polarization perpendicular to the nanowire’s c -axis. Transitions with the light-hole state are always forbidden (indicated by a cross). Full size image Engineering the band structure, so that one or the other conduction band state is lower in energy, would have a major impact on the electronic transport [18] and optical properties of WZ materials. In some III-V alloys, the dark and the bright conduction band are distant in energy and their separation is completely determined by the alloy ionicity [16] , [19] . However, this is not the case for GaAs. After considerable experimental effort [20] , [21] , [22] , [23] , [24] , [25] , measurements were able to precisely define the value of the energy bandgap [14] , [26] , but the energy difference between the two conduction states could not be determined. Indirect measurements merely suggested hints of their energetic proximity [14] . Theoretical investigations addressing this topic have failed to provide a conclusive answer. Some density functional theory studies [16] , [27] predicted a direct bandgap configuration in WZ GaAs, in which the bright conduction band is energetically favoured. Other ab-initio calculations [28] that included spin–orbit interactions predicted a pseudodirect bandgap configuration, in which the dark conduction band has the lowest energy. This band alignment imparts interesting optical properties to WZ crystals: the conduction and valence band wavefunctions have a strong overlap at the Γ-point, but light emission is weak because of symmetry reasons. Further ab-initio calculations, performed on very small nanowires, highlighted the possibility of inducing indirect bandgap configuration in GaAs WZ crystals [29] , [30] . These apparently conflicting theoretical results indicate that the bright and the dark conduction band of WZ GaAs are so close in energy that small perturbations, like a spin–orbit interaction or strain, can switch their order, making this material system an ideal platform to study direct-to-pseudodirect transitions. Studying the effect of uniaxial stress on the light emission of WZ nanowires can clarify their band structure. Because of the large range of elastic deformation of GaAs nanowires [9] , significant energy level shifts and band structure splittings can be induced, enabling us to interpolate and accurately determine the energy difference between the electronic states in unstrained conditions. Optical spectroscopy of WZ nanowires upon uniaxial stress To investigate the direct-to-pseudodirect transition in WZ GaAs upon the application of uniaxial stress, we fabricated free-standing structures by clamping single nanowires to a flexible substrate [31] ( Fig. 2 ). We used single core-shell GaAs-AlGaAs-GaAs nanowires grown along the c -axis (details can be found in the methods section) [14] , [32] . By gradually bending the substrate, in concave or convex manner, a continuous compressive or tensile deformation can be induced on the substrate surface and transferred to the nanowire. Photoluminescence (PL) and Raman spectra were collected at room temperature to obtain information on the band structure and to locally measure the strain applied to the nanowire. 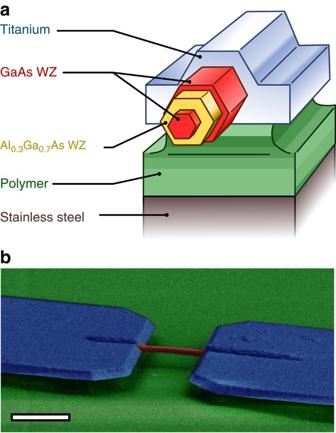Figure 2: Wurtzite GaAs nanowire strain device. (a) Schematic cross-section of a nanowire strain device. A single core-shell WZ GaAs-AlGaAs-GaAs nanowire (GaAs is represented in red, AlGaAs in yellow) is clamped at both ends to a flexible substrate made of stainless steel coated with a transparent polymer (shown in green). Titanium metal clamps (shown in blue) ensure that the nanowire ends are fixed to the substrate. Note that the device dimensions are not to scale. (b) False-colour scanning electron micrograph of a nanowire strain device. The scale bar is 1 μm long. The same colour scheme as inahas been used to identify the various device parts. Figure 2: Wurtzite GaAs nanowire strain device. ( a ) Schematic cross-section of a nanowire strain device. A single core-shell WZ GaAs-AlGaAs-GaAs nanowire (GaAs is represented in red, AlGaAs in yellow) is clamped at both ends to a flexible substrate made of stainless steel coated with a transparent polymer (shown in green). Titanium metal clamps (shown in blue) ensure that the nanowire ends are fixed to the substrate. Note that the device dimensions are not to scale. ( b ) False-colour scanning electron micrograph of a nanowire strain device. The scale bar is 1 μm long. The same colour scheme as in a has been used to identify the various device parts. Full size image The left panel of Fig. 3 shows the Raman spectra measured on a nanowire, plotted as a function of uniaxial stress. The spectra have been acquired by aligning both the laser excitation and the light collected by the spectrometer with polarization parallel to the nanowire axis. This configuration, shown in the inset, minimizes dielectric mismatch effects and ensures the highest optical coupling with the nanowire [33] . The curve in green at the centre of the panel, indicated by the dashed line, was measured without application of stress. Two peaks, namely, the transversal optical (TO) phonon (symmetry A 1 ) and the longitudinal optical (LO) phonon (symmetry E 1 ), are observed at 265.5 cm −1 ±0.3 cm −1 and 289.2 cm −1 ±0.4 cm −1 , respectively. The Raman spectra measured upon application of tensile stress are shown in red in the upper part of the graph, whereas the spectra measured upon compression are shown in blue in the lower part. Both TO and LO phonons experience a linear shift with applied stress. The TO phonon shows the largest energy shift, down to 256.6 cm −1 with tension and up to 272.2 cm −1 with compression. The LO phonon undergoes a more moderate shift, downward in energy to 286.6 cm −1 under tension and upward to 292.2 cm −1 under compression. 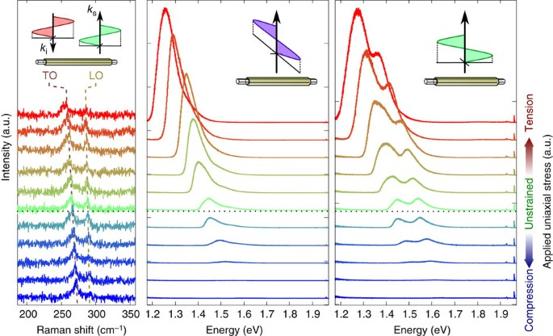Figure 3: Uniaxial stress effects in wurtzite GaAs nanowires. Optical spectra collected from a strained WZ GaAs nanowire. The spectra acquired with increasing tensile stress are shown in red, those acquired with increasing compression in blue. The spectra shown in green close to the dashed line are collected without any strain applied. The Raman spectra are shown in the left panel and have been collected with both the laser and the detector polarization aligned with the nanowire axis (the scattering configuration sketch is shown in the inset). The dotted lines are a guide-to-the-eye to indicate the positions of the phonon peaks attributed to the GaAs transversal optical (TO) phonon with symmetry A1and the longitudinal optical (LO) phonon with symmetry E1. Photoluminescence spectra acquired with polarization orthogonal and parallel to the nanowire axis are shown in the centre and right panel, respectively. The analyser configuration is sketched in the inset of each panel. Figure 3: Uniaxial stress effects in wurtzite GaAs nanowires. Optical spectra collected from a strained WZ GaAs nanowire. The spectra acquired with increasing tensile stress are shown in red, those acquired with increasing compression in blue. The spectra shown in green close to the dashed line are collected without any strain applied. The Raman spectra are shown in the left panel and have been collected with both the laser and the detector polarization aligned with the nanowire axis (the scattering configuration sketch is shown in the inset). The dotted lines are a guide-to-the-eye to indicate the positions of the phonon peaks attributed to the GaAs transversal optical (TO) phonon with symmetry A 1 and the longitudinal optical (LO) phonon with symmetry E 1 . Photoluminescence spectra acquired with polarization orthogonal and parallel to the nanowire axis are shown in the centre and right panel, respectively. The analyser configuration is sketched in the inset of each panel. Full size image In the absence of mechanical buckling (see Supplementary Note 1 and Supplementary Fig. 1 ), the energy shift of the TO and LO phonons are expected to depend linearly [34] on the strain of the nanowire and follow different slopes depending on the direction of atomic displacement, providing information about the strain tensor components [31] . Indeed, the linear dependence between the applied axial strain and the phonon shifts indicates that the nanowire undergoes elastic deformations. However, as no phonon deformation potentials have been determined for WZ GaAs, the peak shifts can only be used to measure the relative strain of the nanowire. The centre and the right panel of Fig. 3 show the PL spectra measured as function of stress with polarization orthogonal and parallel to the nanowire axis, respectively. The spectra acquired without applied uniaxial stress (green curves, close to the dashed line) exhibit two PL peaks at 1.451 eV and 1.544 eV. When the polarizer is oriented orthogonally to the nanowire, the low-energy PL peak has the highest intensity, whereas the high-energy peak contributes a small shoulder. In contrast, if the polarization is oriented parallel to the nanowire, the two peaks have comparable intensities. The spectra acquired upon increasing tension are shown in red, displaced towards the upper part of the plot. The low-energy PL peak shifts by 200 meV towards lower energies. The peak found at higher energy also shifts in the same direction, but its distance to the low-energy peak increases from 93 meV with no stress up to 110 meV under maximum tension. Tensile stress affects also the PL intensity, increasing that of the low-energy peak more than eightfold in both polarizations and that of the high-energy peak up to fivefold. The efficiency of the silicon detector drops dramatically below 1.2 eV, limiting the maximum energy shift and tensile strain detectable in our experiment. We expect that, before the elastic deformation limit of the material is reached, larger shifts towards longer wavelengths can be obtained as we have observed in ZB GaAs nanowires [31] . The PL spectra acquired with increasing compressive stress, shown in blue and displaced towards the bottom of the plot, follow the same trends as observed under tensile stress. The peaks shift towards higher energies above 1.57 eV, whereas their energy separation decreases. The intensity of the two peaks decreases drastically and is suppressed by more than three orders of magnitude across the entire stress range from tension to compression. Hence, in contrast to ZB GaAs [31] , the light emission of WZ GaAs nanowires can be switched on and off through the effect of uniaxial strain. To prove that the PL quenching is induced by the elastic deformation of the nanowire and is completely reversible and reproducible, we measured the PL spectra during a loading–unloading cycle: upon increasing compression the PL intensity could be suppressed and, when returning to the unstrained condition, the light emission could be recovered (details can be found in the Supplementary Note 2 and Supplementary Fig. 2 ). k·p model of the band structure under strain The experimental observations discussed so far can be interpreted by considering jointly the selection rules for the optical transitions, shown in Fig. 1 , and the k·p model, shown in Fig. 4 and discussed in detail in the Methods section. The bright conduction band decreases linearly in energy when tensile stress is applied. The heavy-hole band and the dark conduction band follow the opposite trend and increase their energy with tension. The light- and split-off-hole bands, which share the same symmetry character, undergo nonlinear shifts because of the combined effect of strain and spin–orbit interaction. 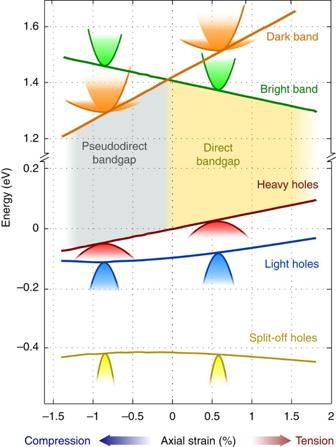Figure 4: k·p model of the uniaxial stress effects in wurtzite GaAs. Heavy holes (in red) with symmetry Γ9vshift linearly towards higher energies when tensile stress is applied. Light holes (shown in blue) and crystal-field split-off holes (shown in yellow) have the same symmetry Γ7v, are coupled by the spin–orbit interaction and undergo nonlinear shifts. In the conduction band, the bright band (symmetry Γ7c, in green) shifts linearly towards lower energies because of the isotropic component of tensile strain. We predict that this band is lowest in energy when no stress is applied. The dark conduction band (symmetry Γ8c, in orange) shifts under stress but in opposite direction of the bright conduction band. The nanowire band structure has a direct bandgap configuration (shaded area in yellow) when the bright conduction band has the lowest energy, and a pseudodirect bandgap configuration (shaded area in grey) when the dark conduction band is lowest. The direct-to-pseudodirect transition occurs when compressive stress is higher than 0.12%. The band structure parameters used in the model were extracted from the fitting shown inFig. 6. Figure 4: k·p model of the uniaxial stress effects in wurtzite GaAs. Heavy holes (in red) with symmetry Γ 9 v shift linearly towards higher energies when tensile stress is applied. Light holes (shown in blue) and crystal-field split-off holes (shown in yellow) have the same symmetry Γ 7 v , are coupled by the spin–orbit interaction and undergo nonlinear shifts. In the conduction band, the bright band (symmetry Γ 7 c , in green) shifts linearly towards lower energies because of the isotropic component of tensile strain. We predict that this band is lowest in energy when no stress is applied. The dark conduction band (symmetry Γ 8 c , in orange) shifts under stress but in opposite direction of the bright conduction band. The nanowire band structure has a direct bandgap configuration (shaded area in yellow) when the bright conduction band has the lowest energy, and a pseudodirect bandgap configuration (shaded area in grey) when the dark conduction band is lowest. The direct-to-pseudodirect transition occurs when compressive stress is higher than 0.12%. The band structure parameters used in the model were extracted from the fitting shown in Fig. 6 . Full size image When tensile stress is applied to the nanowire, the bright conduction band becomes energetically favourable, and electronic transitions towards both the heavy- and light-hole bands can occur with high oscillator strength. The low-energy PL peak (1.451 eV under zero stress) can be attributed to the transitions between the bright conduction band and the heavy-hole band. These photons are highly polarized in the direction orthogonal to the nanowire axis, as expected from the model shown in Fig. 1 . In contrast, the high-energy photons (1.544 eV under zero stress) are generated by transitions between the bright conduction band and the light-hole band and, as expected, have a strong polarization component aligned in the same direction as the nanowire axis. When increasing tensile stress is applied, the energy difference between the heavy- and light-hole band edges increases, holes tend to populate the heavy-hole states with higher density, and the intensity of the corresponding PL peak becomes larger. However, the optical coupling of such photons to the environment is low because of dielectric mismatch effects [33] . Because of this bottleneck, holes populate also the light-hole band and, by recombining with electrons of the bright conduction band, generate photons polarized along the nanowire axis, which are not damped by dielectric mismatch effects. When increasing compressive stress is applied to the nanowire, the dark conduction band becomes energetically favourable, achieving a pseudodirect bandgap configuration. The electrons populate these states with high density, but cannot easily recombine towards any valence band state. Optical transitions from this band towards the heavy-hole band can occur with polarization perpendicular to the nanowire’s c -axis, but have only small oscillator strength. All other transitions are completely forbidden [35] . When the dark conduction band decreases in energy, below the bright conduction band minimum, the PL intensity decreases accordingly. Optical transitions in the pseudodirect configuration To investigate the weak PL generated by the visible optical transitions in the pseudodirect bandgap configuration, we plot in Fig. 5 the intensity of the PL spectra normalized to unity and acquired with the uniaxial stress conditions ranging from unstrained (green data points) to compressive (blue data points). With increasing compression, the PL peaks shift towards high energy, as in Fig. 3 . However, as soon as the low-energy peak reaches 1.47 eV, a shoulder appears around 1.38 eV. If the compressive stress is increased further, this PL component increases in intensity and shifts towards lower energy, exhibiting the opposite trend of that of the other peaks. This PL component is also strongly polarized perpendicularly to the nanowire axis. Both observations are characteristic of a transition between the dark conduction band and the heavy-hole band. To support this interpretation, we fit the PL spectra with line shapes that match the theoretical model shown in Fig. 1 and also follow the colour scheme therein (see Methods section for details). The purple and green peaks correspond to the photons emitted by the transitions between the bright conduction band electrons and heavy holes or light holes, respectively. The red peak corresponds to the transitions between the electronic states of the dark conduction band and heavy holes. A fourth dark transition, whose origin is not yet clear, is shown in yellow. 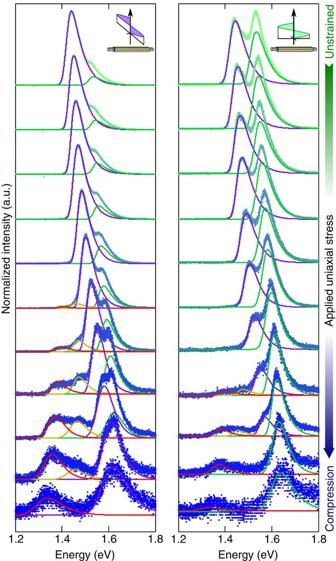Figure 5: Normalized photoluminescence spectra acquired under increasing compression. The normalized PL spectra have been acquired with the polarization perpendicular (left plot) and parallel (right plot) to the nanowire axis. The analyser configurations are sketched in the insets. PL spectra measured without applied stress (data points in green) are plotted on the upper part of each plot, whereas the spectra on the lower part (data points in blue) have been measured under increasing compressive stress. Each spectrum has been fitted using up to four line-shapes, plotted as continuous lines and whose colour code corresponds to the optical transitions shown inFig. 1: transitions from the bright band into heavy- and light-hole states are shown in purple and green, respectively; transitions from the dark conduction band into the heavy-hole band are shown in red. The transitions shown in yellow could not be assigned to any transition involving only states of the GaAs nanowire core. Figure 5: Normalized photoluminescence spectra acquired under increasing compression. The normalized PL spectra have been acquired with the polarization perpendicular (left plot) and parallel (right plot) to the nanowire axis. The analyser configurations are sketched in the insets. PL spectra measured without applied stress (data points in green) are plotted on the upper part of each plot, whereas the spectra on the lower part (data points in blue) have been measured under increasing compressive stress. Each spectrum has been fitted using up to four line-shapes, plotted as continuous lines and whose colour code corresponds to the optical transitions shown in Fig. 1 : transitions from the bright band into heavy- and light-hole states are shown in purple and green, respectively; transitions from the dark conduction band into the heavy-hole band are shown in red. The transitions shown in yellow could not be assigned to any transition involving only states of the GaAs nanowire core. Full size image Estimating strain and band structure parameters The energy difference between conduction and valence band states obtained by such a fitting, extracted from two different nanowire devices (squares and circles), have been plotted in Fig. 6 together with the corresponding TO peak position, which provides a relative measure of the nanowire strain. A low TO phonon energy characterizes a state of tensile strain, whereas a high TO energy corresponds to a state of compression. We fit the joint PL-Raman data points with the stress dependence predicted from the k·p model [36] , [37] shown in Fig. 4 , using the deformation potentials obtained from ab-initio calculations [38] (see Methods section): the result of the fit is plotted with continuous lines in Fig. 6 . This methodology permits us to estimate the axial strain induced in the nanowire as well as the value and the uncertainty of the parameters that define the band structure in unstrained conditions. The range of axial strain is comparable to the one estimated in identical experiments made on ZB nanowire devices with a similar core-shell structure and alloy composition. As the mechanical properties of ZB and WZ crystals are expected to be similar [39] (see Supplementary Note 3 and Supplementary Table 2 ), the excellent agreement between the strain in these two experiments confirms the accuracy of the band-edge deformation potentials used. Although with high uncertainty, the estimated Poisson ratio ν =0.17±0.17 agrees with the value expected (0.188) using Martin’s relations [39] and the elastic properties of bulk GaAs. The optical bandgap of the unstrained nanowire is found to be E gap =1.417 eV±8 meV, in agreement with the value expected [14] at a temperature of 398 K±32 K, which has been estimated from the PL fit (see Methods section). This value is bigger than that of ZB GaAs at the same temperature (1.376 eV±15 meV), in agreement with other experimental results [14] , [26] , [40] . For the first time, we can determine the energy difference between the bright and the dark conduction band in unstrained conditions, which is equal to 33 meV±47 meV: even if only by few tens of meV, the bright conduction band is energetically more favourable in unstrained conditions. The crystal field splitting and spin–orbit splitting of the unstrained nanowires are found to be Δ CR =197 meV±50 meV and Δ SO =293 meV±129 meV, respectively. Both of these values agree well with other experimental results [41] , [42] (Δ SO =379 meV) and theoretical predictions (the crystal field splitting ranges from 180 meV to 212 meV between different ab-initio methods). The WZ GaAs k·p model can therefore explain all optical transitions observed in our experiment, with the exception of the photons identified by the yellow peak in Fig 5 . Further investigations are needed to elucidate the nature of these peaks and are currently ongoing. 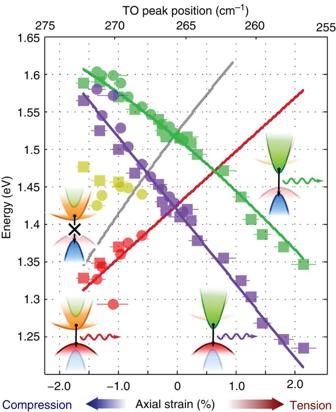Figure 6: k·p model of the uniaxial stress effects in wurtzite GaAs. The energy of the optical transitions, extracted from the fits of the photoluminescence spectra shown inFig. 5, are plotted as a function of the transversal optical (TO) phonon peak position (top abscissa) and of the inferred axial strain (bottom abscissa). The energy uncertainties are smaller than the symbol dimensions. Squares and circles represent the values obtained from two different nanowire devices. The zero-strain position has been identified by measuring the average of the TO peak position (265.5±0.3 cm−1) for three different unclamped nanowires lying on the substrate surface. Continuous lines correspond to the uniaxial strain dependence of the photon energy expected from a k·p model. Following the colour scheme ofFig. 1, we represent the transitions between the bright conduction band and the heavy- and light-hole states in purple and green, respectively. The transitions between the dark conduction band and the heavy-hole band are shown in red, whereas the forbidden transitions between the dark conduction band and the light hole are represented by a grey line. All data points agree very well with the model with the exception of the ones shown in yellow, which follow a nonlinear energy shift that differs between the two nanowire devices. Figure 6: k·p model of the uniaxial stress effects in wurtzite GaAs. The energy of the optical transitions, extracted from the fits of the photoluminescence spectra shown in Fig. 5 , are plotted as a function of the transversal optical (TO) phonon peak position (top abscissa) and of the inferred axial strain (bottom abscissa). The energy uncertainties are smaller than the symbol dimensions. Squares and circles represent the values obtained from two different nanowire devices. The zero-strain position has been identified by measuring the average of the TO peak position (265.5±0.3 cm −1 ) for three different unclamped nanowires lying on the substrate surface. Continuous lines correspond to the uniaxial strain dependence of the photon energy expected from a k·p model. Following the colour scheme of Fig. 1 , we represent the transitions between the bright conduction band and the heavy- and light-hole states in purple and green, respectively. The transitions between the dark conduction band and the heavy-hole band are shown in red, whereas the forbidden transitions between the dark conduction band and the light hole are represented by a grey line. All data points agree very well with the model with the exception of the ones shown in yellow, which follow a nonlinear energy shift that differs between the two nanowire devices. Full size image Checking the consistency of the k·p model To gather further evidence of the accuracy of the k·p model and of the estimation of the band structure parameters E gap , Δ E C , Δ CR and Δ SO evaluated in unstrained conditions, we investigated the strain dependence of the high-energy region of the optical spectra. The energy difference between the bright conduction band and the split-off hole band is in very close proximity to the energy of the laser excitation: these optical transitions are expected to give rise to resonance phenomena or be observed directly. 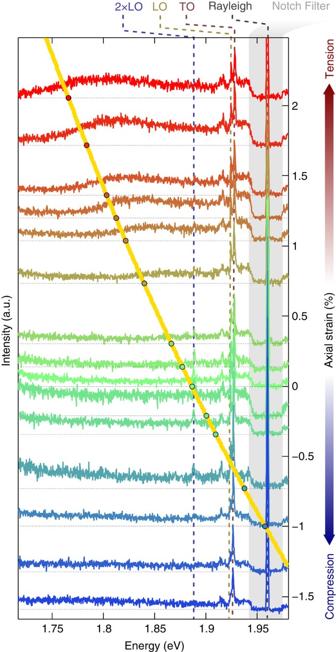Figure 7: Optical spectroscopy fingerprint of the transitions into the split-off hole band. PL and Raman spectra are measured as a function of uniaxial stress in the high-energy region in close proximity of the laser excitation (1.962 eV), with the polarization of the laser excitation and of the detection oriented parallel to the nanowire axis. The spectra are shifted in ordinate to match the value of estimated axial strain and are coloured according to the applied stress as inFig. 3. The energy difference between the bright conduction band and the split-off hole band, as predicted by the k·p model, is shown by a yellow line superimposed onto the PL spectra. Guides to the eye show the position of the Raman peaks assigned to longitudinal optical phonon (LO) overtones, to the transversal optical phonon (TO) peaks as well as the Rayleigh line. Figure 7 shows the high energy region of the optical spectra of WZ GaAs nanowires, measured as a function of uniaxial stress. Indeed, these optical transitions become directly observable in PL at the energy predicted by the model, between 1.72 eV and 1.88 eV, for tensile stress higher than 1.0%. As the light-hole band and crystal-field split-off band share the same symmetry character (Γ 7 v ), we expect the transitions between the bright conduction band and the split-off band to follow the same selection rules as those describing transitions between the bright conduction band and the light-hole band. As expected, the observed PL peaks show a strong polarization parallel to the nanowire axis. For stress values between 0.5% and −1.0%, the optical transitions between the bright conduction band and the split-off band coincide with the laser photon energy (incoming resonance at 1.960 eV) as well as with the scattered photon energy because of the Raman scattering of LO phonons (outgoing resonance around 1.927 eV). Under such resonance conditions, the electron–phonon Fröhlich interaction [43] allows the observation of the LO phonon, which otherwise is not observable in this scattering configuration because of the Raman selection rules [44] . The resonant enhancement can therefore explain the intensity modulation of the LO phonon line observed in the left panel of Fig. 3 . The Fröhlich interaction also enables the scattering of LO overtones visible around 1.888 eV. A similar type of resonant behaviour has already been observed in bulk ZB GaAs [43] . This set of observations provides a further consistency check for the extracted band structure parameters E gap , Δ E C , Δ CR and Δ SO inferred by fitting the experimental data with the k·p model. Figure 7: Optical spectroscopy fingerprint of the transitions into the split-off hole band. PL and Raman spectra are measured as a function of uniaxial stress in the high-energy region in close proximity of the laser excitation (1.962 eV), with the polarization of the laser excitation and of the detection oriented parallel to the nanowire axis. The spectra are shifted in ordinate to match the value of estimated axial strain and are coloured according to the applied stress as in Fig. 3 . The energy difference between the bright conduction band and the split-off hole band, as predicted by the k·p model, is shown by a yellow line superimposed onto the PL spectra. Guides to the eye show the position of the Raman peaks assigned to longitudinal optical phonon (LO) overtones, to the transversal optical phonon (TO) peaks as well as the Rayleigh line. Full size image In conclusion, we performed PL and Raman measurements on single WZ GaAs nanowires under both tensile and compressive uniaxial stress. We demonstrated a remarkable energy shift of the PL because of transitions involving the bright conduction band and, respectively, the heavy-hole band (345 meV) and the light-hole band (257 meV), by varying the strain over a range of ±2%. A direct-to-pseudodirect transition was observed for the first time by a reversible quenching of the PL. The splitting between the dark and bright conduction bands could be tuned continuously over a range of more than 230 meV. Using the Raman scattering spectra as relative strain gauge and fitting the PL energies to a k·p model, we were able to determine all band structure parameters of the WZ GaAs nanowire in unstrained conditions, that is, the crystal field and spin–orbit splitting, the bandgap and, most importantly, the splitting between the bright and the dark conduction bands. Mechanical properties, such as the Poisson ratio of the nanowire, have also been determined. Resonant Raman and the direct optical transitions involving the bright conduction band and the split-off hole band have been investigated and their analysis provided a consistency check of the band structure parameters extracted. The possibility to induce a direct-to-pseudodirect transition in WZ GaAs nanowires—and on other ad-hoc designed WZ III-V alloys—has the potential to be relevant in many optoelectronic applications. On the one end, WZ III-V semiconductors in the pseudodirect bandgap configuration can offer low probability of re-emission processes similar to indirect bandgap materials, which enables to increase the carrier lifetime and the quantum efficiency of photodetectors, as well as decreasing dark currents and generation-recombination noise [45] . On the other end, in the direct bandgap configuration, WZ III-V semiconductors can offer also the high oscillator strength needed for applications that involve light emission. These results pave the way for a new generation of devices that can simultaneously serve as efficient light emitters and efficient photodetectors by leveraging the uniaxial strain degree of freedom. Nanowire growth and characterization GaAs-AlGaAs core-shell nanowires (~40 nm GaAs core, ~40 nm Al 0.3 Ga 0.7 As shell, ~3 nm GaAs shell, ~4 μm long) were grown by the Au-catalysed vapour–liquid–solid method in a molecular beam epitaxy reactor [32] . The nanowire growth direction is parallel to the WZ c -axis. The lattice-matched Al 0.3 Ga 0.7 As shell ensures stable and intense PL of the GaAs core without introducing interfacial strain. The second GaAs shell acts as an oxidation barrier and permits us to perform the optical measurements at room temperature over weeks without any degradation. No strain gradients are expected between the core–shell interfaces (see Supplementary Note 3 ). High-resolution transmission electron micrographs of the nanowires show the WZ structure with a low density of stacking faults [14] . Sample preparation Flexible stainless steel substrates, coated with a transparent polymer, have been used for realizing free-standing, double-clamped nanowire devices [31] . The metal clamps have been fabricated by e-beam lithography and lift-off, using 180 nm of titanium deposited by e-beam evaporation. Reactive ion etching was used to under-etch the polymer to decouple the nanowire from the substrate surface. The free-standing length is 1 μm. Measurement technique To induce uniaxial strain in the nanowire, the underlying sample is bent using a three-point bending mechanism. The mechanism is mounted on the stage of a commercial Raman microscope [31] . This tool has been equipped with two units to enable selection of the polarization orientation of the laser light (excitation path) and of the light collected by the spectrometer (analytic path). Each system consists of one fixed polarizer and a half-wave plate, whose orientation is controlled by a stepper motor. The nanowires have been excited with a low-power He–Ne laser ( P ≤16 μW, λ =632 nm). The light from the nanowire has been collected using a 100x long-working distance objective (working distance of 3.4 mm, numerical aperture of 0.8) and detected by a liquid-nitrogen-cooled silicon charge-coupled device. A 1,800 lines per mm grating has been used to measure the Raman spectra, whereas the PL spectra were measured with a 300 lines per mm grating. Reproducibility The results have been reproduced in more than three different nanowire devices. Figures 3 and 5 show PL spectra measured in two of them. The data extracted from both these measurements have been used in Fig. 6 . Modelling the strain effects in WZ GaAs with the k·p method In the experiment described in this paper, WZ GaAs nanowires are subjected to uniaxial stress parallel to the sixfold symmetry axis ( c -axis). The corresponding strain preserves the symmetry of the unit cell over the entire stress range: the nanowire is elongated along its axis ( ε zz ) and shrinks in the cross-section ( ε xx = ε yy ) because of the finite Poisson ratio ν . The unit cell deformation, shown in Supplementary Fig. 3 , is described by a strain tensor, ε ij , that can be further decomposed in two components: The first term of the sum on the left-hand side of equation (1) represents the isotropic strain component, which causes a variation of the volume of the unit cell but maintains its aspect ratio constant ( c / a ). The second term represents the deviatoric deformation component, which describes the deformation of the unit-cell aspect ratio occurring at constant unit-cell volume. The factor H represents the percentage of isotropic deformation of the unit cell and can be expressed in terms of the Poisson ratio ν by the following relation: Uniaxial strain has a profound impact on the energy levels of the WZ crystals, whose energies can be described accurately using a k·p model. Without applied stress, the band structure is characterized by the bandgap E gap , the conduction band splitting Δ E C , the crystal field splitting Δ CR and the spin–orbit splitting Δ SO . In the framework of the cubic approximation, the strain relation of the energy difference between the valence and conduction band states assumes a simple analytical expression, which depends on few more band structure parameters [36] , [37] : Here E d , E b , E hh , E lh and E so are the energy of the dark and bright conduction bands and of the heavy-hole, light-hole and crystal-field split-off hole bands, evaluated at the Γ-point. The constants Ξ d,h , Ξ b,h and D 1 +2 D 2 are the hydrostatic deformation potentials (in Pikus–Birr notation [36] ) for the dark and the bright conduction band and for the valence band states, whereas Ξ d,u and D 3 are the dark conduction band and the valence band deviatoric deformation potentials. Different ab-initio methods have been used to quantify these constants and provide values, summarized in Supplementary Table 1 , that are robust and consistent within a few percent [38] . Using the relative energy shift of the TO phonon as a relative strain gauge [31] , and fitting the PL shifts with the k·p model shown above, we can identify the unknown quantities ε zz , ν, E gap, Δ E C, Δ CR and Δ SO . Fitting of the PL line-shape We provide in Supplementary Fig. 4 an example of the fitting of the PL measured on an unstrained nanowire with polarization parallel to the nanowire axis (raw data are shown as a continuous black line). For each visible transition, we define a bulk-like joint density-of-states (JDOS) contribution that is proportional to the square root of the energy difference to the transition minimum [1] . In this case, we observe two peaks that are assigned to the transitions between the bright conduction band and, respectively, the heavy-hole band (in red) and the light-hole band (in blue). The total JDOS, given by the sum of the two contributions, is populated with a Boltzmann distribution (in green), which contains information about the electronic temperature. The distribution of possible transitions (area shaded in light blue) obtained in this manner is broadened in energy by performing a convolution integral with a Gaussian function (dark yellow curve). Different factors can contribute to such a broadening, such as a finite recombination lifetime, thermal effects or the presence of stacking faults. After providing an initial estimate for the PL intensities, the peak position of each component, the temperature and the broadening (the last two shared for all JDOS functions), we use a least-square fitting algorithm to find the parameters that reproduce the line-shape best (dashed red line). The result of each spectrum fitting provides a line broadening, an effective temperature, as well as the energy and the intensity of each optical transition. The line broadening is in the range between 10 meV and 35 meV, and the effective temperature ranges between 300 K and 480 K over the entire stress range. Such a temperature increase experienced by the WZ GaAs nanowire agrees well with the one measured in identical experiments in ZB GaAs nanowires and has been assigned to laser-induced heating. How to cite this article: Signorello, G. et al. Inducing a direct-to-pseudodirect bandgap transition in wurtzite GaAs nanowires with uniaxial stress. Nat. Commun. 5:3655 doi: 10.1038/ncomms4655 (2014).